Pseudogap phase of cuprate superconductors confined by Fermi surface topology 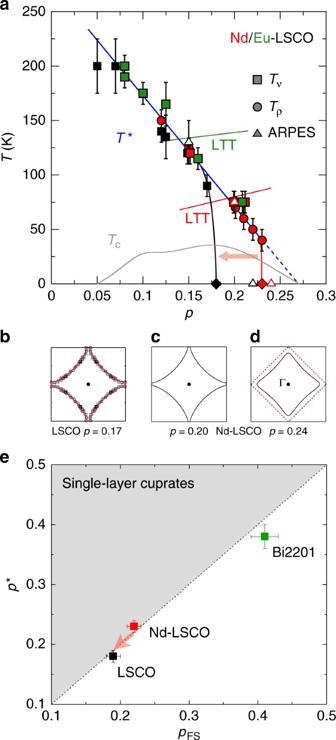Fig. 1 Phase diagram and correlation betweenp* andpFS.aTemperature-doping phase diagram, showing the pseudogap temperatureT* measured by ARPES (triangles), electrical resistivity (circles) and Nernst effect (squares), in LSCO (black), Nd-LSCO (red) and Eu-LSCO (green) (adapted from ref.6; see references therein). The diamonds mark the critical dopingp* at which the pseudogap phase ends atT= 0 (in the absence of superconductivity), for LSCO (black;p* = 0.18, refs.8,9) and Nd-LSCO (red;p* = 0.23, refs.4,5). The short solid lines mark the transition into the low-temperature tetragonal structure (LTT) for Eu-LSCO (green; ref.36and Nd-LSCO (red; ref.34), in the interval where it crossesT*. The grey line is the superconducting critical temperatureTcof LSCO. The dashed line is a linear extension of theT* line (blue). The red arrow illustrates the effect of applying hydrostatic pressure to Nd-LSCO: it shiftsp* down in doping.b,c,dSketch of the Fermi surface in the first Brillouin zone (frame), as measured by ARPES in LSCO (ref.11) atp= 0.17 (b) and in Nd-LSCO (ref.3) atp =0.20 (c) andp =0.24 (d). The red dashed line is the anti ferromagnetic zone boundary (AFZB), which intersects the hole-like Fermi surface of Nd-LSCO atp =0.20, but not its electron-like surface atp =0.24.eCorrelation betweenp* andpFSin single-layer cuprates.p* is measured in the normal state atT =0, by high-field transport in Nd-LSCO (p* = 0.23 ± 0.01, ref.5) and LSCO (p* = 0.18 ± 0.01, refs.8,9), and by high-field NMR in Bi2201 (p* = 0.38 ± 0.02, ref.10).pFSis measured by ARPES in LSCO (pFS= 0.19 ± 0.01, refs.2,11), Nd-LSCO (pFS= 0.22 ± 0.01; ref.3) and Bi2201 (pFS= 0.41 ± 0.02, ref.12). The red arrow shows the effect of applying pressure to Nd-LSCO (red square). We find thatp* andpFSdecrease in tandem, preserving the equalityp* =pFSand thereby showing thatp* is constrained by the conditionp* ≤pFS. The grey shading marks the forbidden region The properties of cuprate high-temperature superconductors are largely shaped by competing phases whose nature is often a mystery. Chiefly among them is the pseudogap phase, which sets in at a doping p * that is material-dependent. What determines p * is currently an open question. Here we show that the pseudogap cannot open on an electron-like Fermi surface, and can only exist below the doping p FS at which the large Fermi surface goes from hole-like to electron-like, so that p * ≤ p FS . We derive this result from high-magnetic-field transport measurements in La 1.6− x Nd 0.4 Sr x CuO 4 under pressure, which reveal a large and unexpected shift of p * with pressure, driven by a corresponding shift in p FS . This necessary condition for pseudogap formation, imposed by details of the Fermi surface, is a strong constraint for theories of the pseudogap phase. Our finding that p * can be tuned with a modest pressure opens a new route for experimental studies of the pseudogap. A central puzzle of cuprate superconductors [1] , the pseudogap is a partial gap that opens in their spectral function, detected most directly by angle-resolved photoemission spectroscopy (ARPES). It opens below a temperature T * that decreases monotonically with increasing hole concentration (doping) p . For example, T * = 130 ± 20 K in La 2- x Sr x CuO 4 (LSCO) at p = 0.15 [2] and T * = 75 ± 5 K in La 1.6− x Nd 0.4 Sr x CuO 4 (Nd-LSCO) at p = 0.20 [3] . Transport properties like the electrical resistivity ρ( T ) and the Nernst coefficient ν( T ) are affected by the opening of the pseudogap and so may be used to detect T *, as previously reported in refs. [4] , [5] and ref. [6] , respectively. In Fig. 1a , we show the temperature-doping phase diagram of LSCO, Nd-LSCO and La 1.8- x Eu 0.2 Sr x CuO 4 (Eu-LSCO). We see that all three materials have the same T * up to p ~0.17, irrespective of their different crystal structures [6] . Indeed, Nernst data [6] show, for example, that T * = 120 ± 10 K at p = 0.15 in both LSCO and Nd-LSCO, whose structure in that part of the phase diagram is orthorhombic, and T * = 115 ± 10 K at p = 0.16 in Eu-LSCO, whose structure in that part of the phase diagram is tetragonal (LTT) (Supplementary Fig. 1 ). In Nd-LSCO and Eu-LSCO, T * decreases linearly all the way from p ~0.08 to p ~0.23 (blue line in Fig. 1a ). On its trajectory, the T * line goes unperturbed through the LTT transition at p ~0.14 for Eu-LSCO (short green line) and at p ~0.19 for Nd-LSCO (short red line). Clearly, the pseudogap mechanism does not care about the crystal structure (Note that it is also robust against disorder [7] ). Fig. 1 Phase diagram and correlation between p * and p FS . a Temperature-doping phase diagram, showing the pseudogap temperature T * measured by ARPES (triangles), electrical resistivity (circles) and Nernst effect (squares), in LSCO (black), Nd-LSCO (red) and Eu-LSCO (green) (adapted from ref. [6] ; see references therein). The diamonds mark the critical doping p * at which the pseudogap phase ends at T = 0 (in the absence of superconductivity), for LSCO (black; p * = 0.18, refs. [8] , [9] ) and Nd-LSCO (red; p * = 0.23, refs. [4] , [5] ). The short solid lines mark the transition into the low-temperature tetragonal structure (LTT) for Eu-LSCO (green; ref. [36] and Nd-LSCO (red; ref. [34] ), in the interval where it crosses T *. The grey line is the superconducting critical temperature T c of LSCO. The dashed line is a linear extension of the T * line (blue). The red arrow illustrates the effect of applying hydrostatic pressure to Nd-LSCO: it shifts p * down in doping. b , c , d Sketch of the Fermi surface in the first Brillouin zone (frame), as measured by ARPES in LSCO (ref. [11] ) at p = 0.17 ( b ) and in Nd-LSCO (ref. [3] ) at p = 0.20 ( c ) and p = 0.24 ( d ). The red dashed line is the anti ferromagnetic zone boundary (AFZB), which intersects the hole-like Fermi surface of Nd-LSCO at p = 0.20, but not its electron-like surface at p = 0.24. e Correlation between p * and p FS in single-layer cuprates. p * is measured in the normal state at T = 0, by high-field transport in Nd-LSCO ( p * = 0.23 ± 0.01, ref. [5] ) and LSCO ( p * = 0.18 ± 0.01, refs. [8] , [9] ), and by high-field NMR in Bi2201 ( p * = 0.38 ± 0.02, ref. [10] ). p FS is measured by ARPES in LSCO ( p FS = 0.19 ± 0.01, refs. [2] , [11] ), Nd-LSCO ( p FS = 0.22 ± 0.01; ref. [3] ) and Bi2201 ( p FS = 0.41 ± 0.02, ref. [12] ). The red arrow shows the effect of applying pressure to Nd-LSCO (red square). We find that p * and p FS decrease in tandem, preserving the equality p * = p FS and thereby showing that p * is constrained by the condition p * ≤ p FS . The grey shading marks the forbidden region Full size image The critical doping p * at which the pseudogap phase comes to an end, however, is material-specific. In LSCO, the linear decrease in T * vs p comes to an end at p * = 0.18 ± 0.01 [8] , [9] . In Nd-LSCO, resistivity measurements [4] , [5] at p = 0.20 and above show that the T * line only comes to an end at p * = 0.23 ± 0.01. Why does T * not continue to track the dashed blue line in Fig. 1 beyond p = 0.17 for LSCO, or beyond p = 0.23 for Nd-LSCO? In Fig. 1e , we plot p * for the three single-layer cuprates LSCO, Nd-LSCO and Bi2201 [10] , as a function of p FS , the doping at which the Fermi surface undergoes a change from hole-like to electron-like as determined by ARPES measurements [2] , [3] , [11] , [12] . Within error bars, we observe that p * = p FS , in other words, it appears that what limits p * is the constraint that the pseudogap cannot open on an electron-like Fermi surface. In the following, we examine whether this connection is accidental or not, by independently probing how p * and p FS evolve under the effect of hydrostatic pressure in Nd-LSCO. With a maximal T c of only 20 K, this cuprate provides a window into the pseudogap phase near its end point at p *, free of superconductivity, down to the T = 0 limit, achieved by applying a magnetic field of 30 T (or greater), whose sole effect is to suppress superconductivity and reveal the underlying normal state (ref. [5] ). Our measurements reveal a large and unexpected downward shift of p * with pressure, which we find to be driven by a corresponding change in p FS , so that the relation p * ≤ p FS is obeyed. This fundamental property has direct and fundamental implications for the mechanism of pseudogap formation. Determination of p * and p FS Our study is based on transport signatures of p * and p FS . We begin with p *. When p < p *, the electrical resistivity ρ ( T ), Nernst coefficient and Hall coefficient R H ( T ) all exhibit large upturns at low temperature [4] , [5] , [6] , [9] —signatures of the pseudogap phase, attributed to a drop in carrier density n from n = 1 + p above p * to n = p below p * [5] , [9] , [13] . In Nd-LSCO at p = 0.20, ARPES sees a gap opening at T* = 75 K (ref. 3 ), precisely the temperature below which the resistivity exhibits an upward deviation from its high- T linear behaviour [4] , [5] . By contrast, at p = 0.24 the three transport coefficients show no trace of any upturn at low T [4] , [5] , [6] , , with the resistivity remaining linear down to T → 0 (Fig. 2a ), consistent with the absence of a gap in ARPES data [3] . Fig. 2 Effect of pressure on Nd-LSCO. Transport properties of Nd-LSCO as a function of temperature, at different dopings as indicated. In a , c and d , grey data are in zero field and coloured data are in magnetic field. a Resistivity of Nd-LSCO at p = 0.22 from ref. [5] (blue) and at p = 0.24 from ref. 4 (red), in H = 33 T and ambient pressure. At p = 0.22, ρ ( T ) is seen to deviate upwards from its linear T dependence at high T (black line) below the onset temperature T * of the pseudogap phase (Fig. 1a ). b Difference between the data and the linear fits of Supplementary Fig. 6 , showing that the onset of the upturn at T * (arrow) is independent of pressure. The sharp kink is due to the structural transition from orthorhombic at high T (LTO) to tetragonal at low T (LTT) (see Fig. 1 ). c Resistivity of Nd-LSCO at p = 0.22 and H = 33 T, at ambient pressure (blue, ref. 5 ) and P = 2.0 GPa (red, this work), with a linear fit (black line) to the P = 2.0 GPa data. d As in c , but for the Hall coefficient R H ( T ). The horizontal dotted line is the value expected from the large hole-like Fermi surface. Coloured dashed lines are a guide to the eye Full size image In Fig. 3 , we reproduce published data [5] for ρ ( T ) (Fig. 3a ) and R H ( T ) (Fig. 3c ) in Nd-LSCO at different dopings. The upturns decrease as p approaches p * from below. We determine p * as the doping where the upturns in ρ ( T ) and R H ( T ) vanish, giving p * = 0.23 ± 0.01 (Fig. 4 ). (Note that at that doping ρ ( T ) displays a slight upturn while R H ( T ) remains flat. This difference comes possibly from the fact that ρ ( T ) is sensitive to the total carrier density while R H ( T ) is balanced by electron- and hole-like contributions, as in the reconstructed Fermi surface just below p * for an anti ferromagnetic scenario [14] . See discussion in ref. [5] ). Fig. 3 Effect of doping and pressure on Nd-LSCO. Comparing the effect of doping on the pseudogap phase in Nd-LSCO (left panels) to the effect of pressure (right panels). a , b Electrical resistivity expressed as Δ ρ = ρ ( T ) − ρ 0 (normalised at 75 K), where ρ 0 is the residual resistivity estimated from a linear fit to ρ ( T ) above T * (ref. [5] ). The values of Δ ρ at T → 0 are plotted vs p in Fig. 4a . a At ambient pressure, for various dopings as indicated, in H = 33 T (data from ref. [5] ). b At p = 0.21, for different pressures as indicated, in H = 33 T. Data at P = 2.0 GPa and H = 0 are also shown (orange), together with a linear extrapolation to T = 0 (black dotted line). c , d Same as in a and b but for the Hall coefficient R H . Light and dark coloured curves are in H = 16 and 33 T, respectively. The values at T → 0, labelled R H (0), are plotted vs p in Fig. 4b . All dashed lines are a guide to the eye Full size image Fig. 4 Effect of pressure on p *. a Magnitude of the upturn in ρ ( T ) at T → 0 and for H = 33 T as a function of doping, for ambient pressure (blue), P = 1.0 (purple) and 2.0 GPa (red), obtained from ambient pressure data (Fig. 3a ) and from pressure data at p = 0.21 (Fig. 3b ), p = 0.22 (Fig. 2c ) and p = 0.23 (Supplementary Fig. 7 ). The pseudogap critical point p * is where the upturn goes to zero (arrow). b R H (0) vs doping for ambient pressure (blue), P = 1.0 (purple) and 2.0 GPa (red), obtained from ambient pressure data at p = 0.21, 0.22 and 0.23 (Fig. 3c ) for H = 33 T, and p = 0.25 (Supplementary Fig. 4 ) for H = 16 T, and from pressure data at p = 0.21 (Fig. 3d ) and p = 0.22 (Fig. 2d ) for H = 33 T, and p = 0.25 (Supplementary Fig. 4 ) at H = 16 T. All lines are a guide to the eye. The effect of pressure is to shift p * down in doping (grey arrows), by roughly dp * = −0.02 for 2.0 GPa. All the error bars reflect the uncertainty on the extrapolation to T = 0 Full size image We now turn to p FS . In a single-layer cuprate, the Fermi surface changes topology from hole-like at p < p FS (Fig. 1c ) to electron-like at p > p FS (Fig. 1d ). ( p FS is the doping at which the van Hove singularity in the density of states crosses the Fermi level.) ARPES studies show that the Fermi surface is hole-like in LSCO at p = 0.17 [11] and Nd-LSCO at p = 0.20 [3] , while it is electron-like at p = 0.20 [2] and p = 0.24 [3] , respectively, so that p FS = 0.19 ± 0.01 in LSCO and p FS = 0.22 ± 0.01 in Nd-LSCO. Changes under hydrostatic pressure We now examine the effect of pressure on p FS and p *. Pressure is known to change the crystal structure of Nd-LSCO from LTT at ambient pressure to HTT at P > 4.2 GPa [15] . Our band–structure calculations based on a standard tight-binding model (see 'Methods' section and Supplementary Fig. 2 ) show that this causes a decrease in the ratio | t ’/ t |, where t and t ’ are nearest- and next-nearest-neighbour hopping parameters. It is a property of this model that the Fermi surface goes from hole-like to electron-like with decreasing | t ’/ t | (at fixed p ), consistent with fits to ARPES data on LSCO [2] , [11] . Pressure applied to Nd-LSCO is therefore expected to reduce p FS (Fig. 5c ). Although the maximum pressure in our experiment is 2.0 GPa, it still reduces the CuO 6 octahedron tilt angle of the LTT structure significantly towards the HTT phase [15] , which decreases | t ’/ t |. Fig. 5 Effect of pressure on p FS . a Pressure dependence of the Hall coefficient in Nd-LSCO at p = 0.25 > p *, normalised by its value at ambient pressure, R H (0) = 0.4 mm 3 C −1 (Supplementary Fig. 4 ). The dashed line is a linear fit through the data at low pressure, whose slope is −6 % GPa −1 . b Sketch of the doping dependence of R H in LSCO (Supplementary Fig. 3 ), normalised by its value at p FS (blue line). The red line illustrates the effect of shifting p FS down in doping by an amount δ p FS = −0.02 (grey arrow): R H decreases by ~13 % (red arrow). This is the amount by which R H decreases in Nd-LSCO under 2.0 GPa, for p > p * ( a ). c Sketch of the theoretical dependence of p FS on the band–structure parameter t ’/ t . For a given value of t ’/ t , p FS is given by the blue line, which separates the regions where the cuprate Fermi surface is electron-like (above) and hole-like (below). Our band–structure calculations for Nd-LSCO yield t ’/ t = −0.171 in the LTT structure (black) and t ’/ t = −0.152 in the HTT structure (red) (Supplementary Fig. 2 ), so that p FS is expected to decrease (grey arrow) under pressure, as observed experimentally Full size image Experimentally, we study the pressure dependence of p FS by looking at R H for p ≥ p *. In LSCO in the regime above p FS ~0.19, R H decreases linearly with doping as the system moves away from p FS (Supplementary Fig. 3 ), to eventually become negative above p ~0.35 [16] , [17] . Quantitatively, an increase in doping by δ p = 0.02 corresponds to a ~13% drop in R H (Fig. 5b ). Since all there is in this regime is a single large electron-like Fermi surface, Nd-LSCO in the regime above p FS ~0.22 must display a similar linear decrease of R H with doping, possibly with a different absolute value. Hence, the same relative change in R H is expected to correspond to a similar displacement in doping. In Fig. 5a (see also Supplementary Fig. 4 ), we see that R H in Nd-LSCO at p = 0.25 decreases by ~12% under 2 GPa, which implies that p FS in Nd-LSCO shifts down by δ p FS ~0.02 under 2 GPa, based on the LSCO data. To study the pressure dependence of p *, we measured the high-field normal-state resistivity under pressure up to 2 GPa. Our data on LSCO below p * show that the pseudogap is unaffected by pressure, in the sense that the amplitude of the low- T upturn in the resistivity at p = 0.143 (ref. [9] ) is unchanged (Supplementary Fig. 5 ). In Nd-LSCO at p = 0.15, our measurements (Fig. 2b and Supplementary Fig. 6 ) also show that T * is independent of pressure, as previously observed in YBa 2 Cu 3 O y (ref. [18] ). So a pressure of 2 GPa does not tune T * directly. Nevertheless, in Nd-LSCO just below p * we observe a dramatic effect of pressure on the pseudogap: at p = 0.22, 2.0 GPa completely eliminates the low- T upturn in the resistivity (Fig. 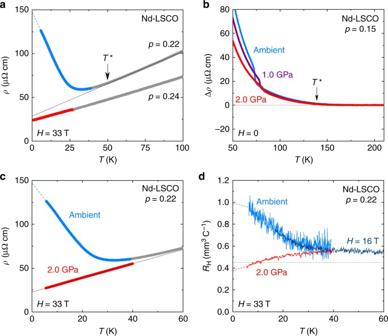Fig. 2 Effect of pressure on Nd-LSCO. Transport properties of Nd-LSCO as a function of temperature, at different dopings as indicated. Ina,candd, grey data are in zero field and coloured data are in magnetic field.aResistivity of Nd-LSCO atp= 0.22 from ref.5(blue) and atp= 0.24 from ref.4(red), inH= 33 T and ambient pressure. Atp= 0.22,ρ(T) is seen to deviate upwards from its linearTdependence at highT(black line) below the onset temperatureT* of the pseudogap phase (Fig.1a).bDifference between the data and the linear fits of Supplementary Fig.6, showing that the onset of the upturn atT* (arrow) is independent of pressure. The sharp kink is due to the structural transition from orthorhombic at highT(LTO) to tetragonal at lowT(LTT) (see Fig.1).cResistivity of Nd-LSCO atp= 0.22 andH= 33 T, at ambient pressure (blue, ref.5) andP= 2.0 GPa (red, this work), with a linear fit (black line) to theP= 2.0 GPa data.dAs inc, but for the Hall coefficientRH(T). The horizontal dotted line is the value expected from the large hole-like Fermi surface. Coloured dashed lines are a guide to the eye 2c ), resulting in a linear T behaviour characteristic of the regime at p * and above (refs. [4] , [8] ). A suppression of the low- T upturn is also seen at p = 0.21 (Fig. 3b ). This large and unexpected effect of pressure on the pseudogap is our main experimental finding. In Fig. 3 , we compare the effect of pressure on the resistivity and Hall coefficient of Nd-LSCO with the effect of doping. (Note that unlike for YBa 2 Cu 3 O y , pressure does not change the doping in Nd-LSCO, which is set by the Sr content.) We see that pressure has the same effect as doping, consistent with a lowering of p * induced by pressure. Quantitatively, p * moves down from 0.23 at P = 0 to 0.21 at P = 2.0 GPa (Fig. 4 ). A downward shift δ p * = −0.02 in 2.0 GPa is the same shift (δ p FS ~ −0.02) that is observed for p FS . We infer that it is the downward movement of p FS that constrains p * to move down with pressure, thereby showing that the condition p * ≤ p FS must hold. This elucidates why the pseudogap phase of LSCO ends at a lower doping than in Nd-LSCO, for indeed p * = p FS in LSCO, within error bars (Fig. 1e ). In most cuprates, p FS is much higher, as in the single-layer material Bi2201, for example, where p FS = 0.41 ± 0.02 (ref. [12] ). Remarkably, p * is nearly as high, with p * = 0.38 ± 0.02 in Bi2201 (ref. [10] ), as illustrated in Fig. 1e . Our finding that p * ≤ p FS is consistent with the known properties of all cuprates. In particular, it holds true for all known single-layer cuprates, including not only those in Fig. 1e , but also Tl 2 Ba 2 CuO 6+δ , for example, where at p ~0.3 the Fermi surface is hole-like and there is no pseudogap [19] . It also holds for bi-layer cuprates, such as Bi 2 Sr 2 CaCu 2 O 8+δ , in the sense that the pseudogap opens only once [20] or after [21] both Fermi surfaces (bonding and anti-bonding) have become hole-like [22] . The close proximity of p * to a van Hove singularity (at p FS ) may have some impact on the physics of the pseudogap. However, since the velocity vanishes at the van Hove point, we do not expect any singularity in the transport properties. Moreover, in the presence of substantial c -axis dispersion, of the order of t z ~20 meV in Nd-LSCO, the divergence in the density of states gets cut off at low temperature [23] . It is striking that a minute change in the Fermi surface, smaller than that illustrated between Fig. 1c ( p slightly below p FS ) and Fig. 1d ( p slightly above p FS ), can switch off a gap of magnitude ~20 meV (ref. [3] ). This extreme sensitivity of the pseudogap on the details of the Fermi surface suggests that for the pseudogap to form it is necessary that the Fermi surface intersects the anti ferromagnetic zone boundary (AFZB), the dashed line in Fig. 1d , as proposed in refs. [20] , [24] . This is precisely what happens when the doping drops below p FS . There is empirical evidence that this intersection may indeed be a crucial element of the pseudogap mechanism. First, this AFZB is where in k -space the separation of ungapped and (pseudo)gapped states occurs, as detected by quasiparticle interference in scanning tunnelling microscopy [21] . In other words, the AFZB is the pseudogap phase’s organising principle in k -space: it defines the so-called 'Fermi arcs'. Note thatwhen the pseudogap turns on (with decreasing T or p ), the k -space area contained by the ungapped states (between the Fermi arcs and the AFZB) goes from A ~ 1 + p to A ~ p (ref. [21] ). Second, upon crossing p * from above, the carrier density measured by the Hall number goes from n = 1 + p to n = p (refs. [5] , [13] ), consistent with A ~ n . The simplest way to obtain a loss of 1.0 hole per planar Cu atom is to reconstruct the large hole-like Fermi surface (with 1 + p holes) by folding it about the AFZB, which produces four small nodal hole pockets (with p holes) [14] . This can be achieved either by AF order with a wavevector Q = ( π , π ) or by an Umklapp surface coincident with the AFZB, as in the YRZ model [25] . If this is indeed how the pseudogap phase transforms the Fermi surface, then no Fermi arcs (or nodal pockets) can form when p > p FS . Electron-doped cuprates provide a clear example of Fermi surface reconstruction caused by long-range AF order, where the AFZB plays a key role, but where no pseudogap phase forms [26] . The issue of why there is a pseudogap in hole-doped cuprates and not in electron-doped cuprates, however, is an open question. If the pseudogap phase needs states near ( π , 0) to form, the question is at what energy do those states have to be relative to ε F ? We presume that they should be within the pseudogap energy Δ PG of ε F . This implies that for p just above p FS , the pseudogap phase can still form. This introduces some 'width' to the criterion p * ≤ p FS . In a similar vein, a 3D dispersion of the Fermi surface in the k z (or c ) direction will also give some 'width' to the criterion, since at a given doping the Fermi surface can be electron-like at some k z value but still hole-like at some other k z value. 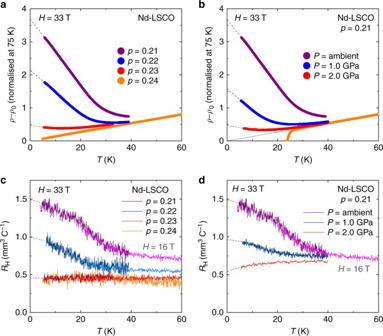Fig. 3 Effect of doping and pressure on Nd-LSCO. Comparing the effect of doping on the pseudogap phase in Nd-LSCO (left panels) to the effect of pressure (right panels).a,bElectrical resistivity expressed as Δρ=ρ(T) −ρ0(normalised at 75 K), whereρ0is the residual resistivity estimated from a linear fit toρ(T) aboveT* (ref.5). The values of ΔρatT→ 0 are plotted vspin Fig.4a.aAt ambient pressure, for various dopings as indicated, inH= 33 T (data from ref.5).bAtp= 0.21, for different pressures as indicated, inH= 33 T. Data atP= 2.0 GPa andH= 0 are also shown (orange), together with a linear extrapolation toT= 0 (black dotted line).c,dSame as inaandbbut for the Hall coefficientRH. Light and dark coloured curves are inH= 16 and 33 T, respectively. The values atT→ 0, labelledRH(0), are plotted vspin Fig.4b. All dashed lines are a guide to the eye The requirement that a pseudogap cannot form in a cuprate with an electron-like Fermi surface imposes a stringent constraint on theories of the pseudogap phase [25] , [27] , [28] , [29] , [30] , [31] . In the YRZ model [25] , a pseudogap forms because carriers undergo Umklapp scattering, inherited from the Mott insulator, at points where the Fermi surface intersects the AFZB; this model therefore agrees with our proposed constraint. Our findings are also broadly consistent with spin-fermion models that hinge on the hot spots that lie at the intersection of Fermi surface and AFZB [27] , [28] . More specifically, two recent theoretical studies [29] , [32] find that a pseudogap only opens on hole-like Fermi surfaces and that p * ≤ p FS for a wide range of band–structure parameters, even in the strong-coupling regime where the anti ferromagnetic correlations responsible for the pseudogap are short ranged. On the other hand, in scenarios characterised by a wavevector Q = (0, 0), the AFZB plays no special role and there is then no obvious reason for the constraint to be effective. This would seem to rule out nematic order [31] and intra-unit cell magnetic order [30] , [33] as possible drivers of the pseudogap phase. Instead, these orders would be secondary instabilities [6] . On the experimental side, the ability to continuously suppress and restore the pseudogap with pressure in a given sample without changing the doping or disorder level provides a promising avenue to study the pseudogap state, compatible with a range of probes such as Raman, optics, X-ray and neutron scattering. LSCO samples Single crystals of La 2− x Sr x CuO 4 (LSCO) were grown by the flux-zone technique, with nominal Sr concentrations of x = 0.145 at Hokkaido University and x = 0.18 at the University of Tokyo. Samples for resistivity measurements were cut in the shape of small rectangular platelets, of typical dimensions 1 mm × 2 mm × 0.5 mm, with the smallest dimension along the c axis. Contacts were made using H20E silver epoxy, diffused by annealing. The hole concentration (doping) p for our nominal x = 0.145 sample was determined using the doping dependence of the (tetragonal to orthorhombic) structural transition temperature, T LTO , which is detected in the resistivity as a small but sharp kink. This yields p = 0.143 (ref. [9] ). For our sample with x = 0.18, we take p = x . Nd-LSCO samples Single crystals of La 2− y − x Nd y Sr x CuO 4 (Nd-LSCO) were grown at the University of Texas at Austin with a Nd content y = 0.4, using a travelling-float-zone technique, and cut from boules with nominal Sr concentrations x = 0.15, 0.21, 0.22, 0.23 and 0.25. The samples were prepared for transport measurements as described above for the LSCO samples. For all five samples, the hole concentration p is given by p = x , with an error bar ±0.003. The samples labelled here p = 0.21, 0.22, 0.23 and 0.24 are the same samples as those studied in ref. [5] ; the sample labelled here p = 0.25 is a new sample, with p = 0.25 ± 0.003. Resistivity and Hall measurements The electrical transport measurements were performed via a standard four-point low AC technique using an SR830 lock-in amplifier and a Keithley 6221 current source. A current of typically 2 mA was applied within the CuO 2 planes and the magnetic field along the c -axis. The longitudinal and Hall resistances R xx and R xy were measured at Sherbrooke in steady fields up to 16 T and at the NHMFL in steady fields up to 45 T. The Hall resistance R xy is obtained by reversing the field and anti-symmetrizing the data, as R xy ( H ) = ( R xy ( + H ) − R xy (− H ))/2. Application of pressure Pressure was applied on our samples using a miniature non-magnetic piston-cylinder cell. The pressure medium is Daphne oil 7474, which remains liquid at all pressures measured here at 300 K, ensuring a high degree of hydrostaticity. The internal pressure is measured both at room temperature and at 4.2 K, using either the fluorescence of a small ruby chip or a Sn manometer. The values quoted throughout are the low temperature pressures. The error bar on all the pressure values is ± 0.05 GPa, which comes from the uncertainty in measuring the position of the fluorescence peaks. For each measurement, the cell was cooled slowly (<1 K min −1 ) to ensure a homogeneous freezing of the pressure medium. Band–structure calculations Band–structure calculations were performed by using the full potential augmented plane wave band method, implemented in the WIEN2k package. We used the local density approximation for the exchange-correlation potential. We used 1000 k-points inside the first Brillouin zone. The convergence of total energy with respect to the number of k-points was checked to have a precision better than 0.007 eV per formula unit. We calculated the electronic structure of La 2 CuO 4 using the structural parameters of Nd-LSCO measured experimentally by X-ray diffraction for both ambient pressure (LTT structure; ref. [34] and P = 4.2 GPa (HTT structure; ref. [15] ). In the case of P = 4.2 GPa (HTT), in order to determine the internal position of atoms inside the CuO 6 octahedron, we assumed an isotropic contraction of the CuO 6 octahedra from hydrostatic pressure. 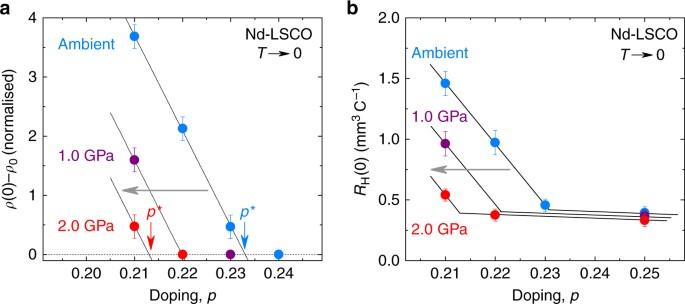Fig. 4 Effect of pressure onp*.aMagnitude of the upturn inρ(T) atT→ 0 and forH= 33 T as a function of doping, for ambient pressure (blue),P= 1.0 (purple) and 2.0 GPa (red), obtained from ambient pressure data (Fig.3a) and from pressure data atp= 0.21 (Fig.3b),p= 0.22 (Fig.2c) andp= 0.23 (Supplementary Fig.7). The pseudogap critical pointp* is where the upturn goes to zero (arrow).bRH(0) vs doping for ambient pressure (blue),P= 1.0 (purple) and 2.0 GPa (red), obtained from ambient pressure data atp= 0.21, 0.22 and 0.23 (Fig.3c) forH= 33 T, andp= 0.25 (Supplementary Fig.4) forH= 16 T, and from pressure data atp= 0.21 (Fig.3d) andp= 0.22 (Fig.2d) forH= 33 T, andp= 0.25 (Supplementary Fig.4) atH= 16 T. All lines are a guide to the eye. The effect of pressure is to shiftp* down in doping (grey arrows), by roughlydp* = −0.02 for 2.0 GPa. All the error bars reflect the uncertainty on the extrapolation toT= 0 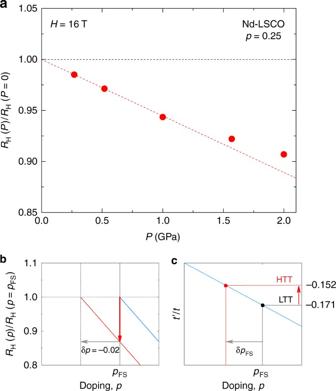Fig. 5 Effect of pressure onpFS.aPressure dependence of the Hall coefficient in Nd-LSCO atp= 0.25 >p*, normalised by its value at ambient pressure,RH(0) = 0.4 mm3C−1(Supplementary Fig.4). The dashed line is a linear fit through the data at low pressure, whose slope is −6 % GPa−1.bSketch of the doping dependence ofRHin LSCO (Supplementary Fig.3), normalised by its value atpFS(blue line). The red line illustrates the effect of shiftingpFSdown in doping by an amount δpFS= −0.02 (grey arrow):RHdecreases by ~13 % (red arrow). This is the amount by whichRHdecreases in Nd-LSCO under 2.0 GPa, forp > p* (a).cSketch of the theoretical dependence ofpFSon the band–structure parametert’/t. For a given value oft’/t,pFSis given by the blue line, which separates the regions where the cuprate Fermi surface is electron-like (above) and hole-like (below). Our band–structure calculations for Nd-LSCO yieldt’/t= −0.171 in the LTT structure (black) andt’/t= −0.152 in the HTT structure (red) (Supplementary Fig.2), so thatpFSis expected to decrease (grey arrow) under pressure, as observed experimentally Experiments on La 2 CuO 4 have shown this assumption to be valid [35] . Tight-binding hopping parameters were obtained by fitting Cu(d x 2- y 2 )-driven bands for high-symmetry points of the anti ferromagnetic zone boundary. Sample size No statistical methods were used to predetermine sample size. Data availability All relevant data are available from the authors.